Three-dimensionally bonded spongy graphene material with super compressive elasticity and near-zero Poisson’s ratio It is a challenge to fabricate graphene bulk materials with properties arising from the nature of individual graphene sheets, and which assemble into monolithic three-dimensional structures. Here we report the scalable self-assembly of randomly oriented graphene sheets into additive-free, essentially homogenous graphene sponge materials that provide a combination of both cork-like and rubber-like properties. These graphene sponges, with densities similar to air, display Poisson’s ratios in all directions that are near-zero and largely strain-independent during reversible compression to giant strains. And at the same time, they function as enthalpic rubbers, which can recover up to 98% compression in air and 90% in liquids, and operate between −196 and 900 °C. Furthermore, these sponges provide reversible liquid absorption for hundreds of cycles and then discharge it within seconds, while still providing an effective near-zero Poisson’s ratio. Graphene sheets and carbon nanotubes (CNTs) possess extraordinary flexibility and strength and can be assembled into very low-density, three-dimensional (3D) structures that are highly elastomeric [1] , [2] , [3] , [4] , [5] , [6] , [7] , [8] , [9] . In particular, aerogels exhibiting reversible strains of 50–90% have been synthesized from graphene oxide (GO) mixed with materials that influence compressibility, such as CNTs [2] , [3] , polypyrrole [4] , ethylenediamine [5] and polyurethane [6] . Additive-free, highly anisotropic graphene aerogels that can withstand repeated 80% compression have been reported and it shows an anisotropic structure [7] . But it is still a great challenge to fabricate graphene-only bulk materials with its unique properties arising from the nature of individual graphene sheets and the monolithic 3D structures these sheets might be able to assemble into. On the other hand, while cork has near-zero Poisson’s ratio in one direction, it does not demonstrate good elastic performance. In this work, we describe a unique bulk and monothlic grapheme-based sponge material, synthesized by a modified solvothermal reaction of GO sheets in alcohol and a subsequent thermal annealing to provide GO reduction and desired restoration of the graphene intrinsic structure and properties, which exhibits both superelastic performance like rubber and near-zero Poisson’s ratio in all directions like cork. These sponges have air-like densities and demonstrate highly repeatable compression and complete recovery in a wide temperature in air and liquid without substantial degradation. Furthermore, reversible rubber-like compressive elasticity was observed even in extreme environments, such as in liquid nitrogen (−196 °C) and at temperatures as high as 900 °C. Even when the maximum (>99%) strain is applied, the graphene sponge exhibits highly repeatable compression reversibility. Dynamic mechanical analysis (DMA) measurements demonstrate that the storage and loss moduli of our sponges are largely independent of temperature and frequency, indicating that the origin of elasticity is enthalpic (rather than entropic, as for ordinary rubbers) [10] , [11] . Furthermore, the graphene sponge that absorbs over 1,000 times its weight in pump oil, and reversibly discharges a similar amount during subsequent compression. More importantly, these graphene sponges display a near-zero Poisson’s ratio in all directions in both air and liquids, which means that compression does not significantly change their dimensions at the perpendicular directions. This appears to be the first reported carbon aerogel that isotropically combines, for all strains, the near-zero Poisson’s ratio of cork (which only applies in the cork’s axial direction) [12] with the high-strain compressive elasticity of a rubber. The combination of characteristic and exclusive properties from cork and rubber observed for this material in a wide temperature range and in air and liquids, indicate that this material may have a great potential for some novel applications when multifold properties are needed. This also demonstrates that if 2D materials are assembled into 3D mode where the properties of such 2D building blocks are kept, novel and combined properties may be observed. Synthesis Our method for graphene sponge synthesis, detailed in the Supplementary Methods used a modified conventional hydrothermal method [13] , [14] , thereby yielding new combinations of graphene sponge properties. In brief, GO sheets ( Supplementary Fig. 1 ) are first solvothermally assembled in ethanol to obtain a nearly homogenous, ethanol-filled material ( Fig. 1a ). Following a slow exchange of ethanol with water, the sponge is freeze-dried and then annealed under inert atmosphere at 400 °C to obtain the final graphene sponge [15] ( Fig. 1b ). Importantly, the size of GO sheets has a great impact on the product’s mechanical properties, and the optimized materials and results are obtained when large size (tens of μm lateral dimension) GO were used. 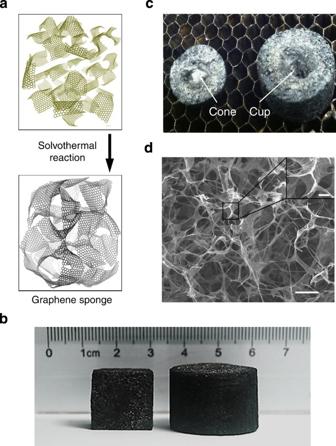Figure 1: The synthesis and structure of graphene sponges. (a) Illustration of the solvothermal conversion of ethanol-dispersed GO platelets into a graphene sponge. (b) Photographs of rectangular (left) and cylindrical (right) graphene sponges. (c) An optical image of the cup and cone structure that is observed when the graphene sponge is elongated to fracture. Scale bar, 1 cm. (d) A radial cross-sectional SEM image of a graphene sponge (scale bar, 20 μm) and a magnified SEM image (inset, scale bar, 5 μm) showing an interwall connection. Figure 1: The synthesis and structure of graphene sponges. ( a ) Illustration of the solvothermal conversion of ethanol-dispersed GO platelets into a graphene sponge. ( b ) Photographs of rectangular (left) and cylindrical (right) graphene sponges. ( c ) An optical image of the cup and cone structure that is observed when the graphene sponge is elongated to fracture. Scale bar, 1 cm. ( d ) A radial cross-sectional SEM image of a graphene sponge (scale bar, 20 μm) and a magnified SEM image (inset, scale bar, 5 μm) showing an interwall connection. Full size image The condensation/cross-linking of the functional groups during synthesis, such as OH, COOH and epoxy groups that are mainly located on GO sheets edges, is expected to covalently interconnect the sheets, thereby forming a monolithic 3D chemically linked network [13] , [16] , [17] , though no direct evidence is available yet. The subsequent annealing step would remove most of the functional groups, partially restoring π-conjugation and increasing electrical conductivity [18] , [19] . By varying the GO concentrations used for the solvothermal reaction, graphene sponges possessing densities from 0.3 to 14 mg cm −3 were obtained, which in the former case have a much lower density than ambient air (1.2 mg cm −3 ). Unless otherwise noted, the results discussed below are for sponges having an uncompressed density of 0.9–2.0 mg cm −3 , though different samples tested with the above density range gave similar results in terms of super compressive elasticity and near-zero Poisson’s ratio. Structure and morphology analysis Elemental analysis shows that our graphene sponge contains ~86 wt% C, ~12 wt% O and ~1–2 wt% H. X-ray photoelectron spectroscopy studies ( Supplementary Fig. 2 ) indicate the existence of ether C–O (~286.7 eV) and ester C(=O)O (~288.6 eV) bonds, in addition to the dominant C=C bonds (~284.5 eV [20] ). Under present solvothermal synthesis conditions, reactions are expected [14] , [21] between/among the OH, COOH and epoxy bond functional groups of adjacent graphene sheets to generate aromatic ether and ester bonds between the sheets mainly at the edges [13] , [16] , [17] . The existence of a significant amount of C–O carbon (~3.7 at%), C=O carbon (~1.6 at%) and C(=O)O ester carbonyl carbon (~1.7 at%) is consistent with the observed corresponding peak for the C–O bonds in infrared spectra ( Supplementary Fig. 3 ) [22] and the enhanced oxygen atom density in regions connecting graphene sheets, which is seen by energy-filtering transmission electron microscopy mapping ( Supplementary Fig. 4 ) [23] . Though there is no direct evidence, this possible bonding between graphene sheets is further suggested by the observation of a ductile cup and cone tensile fracture ( Fig. 1c ) [24] , [25] , the mechanical robustness of the sponges when reversibly compressed and the retention of highly structural stability and large-strain elasticity to at least 900 °C. Also, if there is no strong force to hold the graphene sheets together, it is expected that this bulk material would just collapse or fall apart at extreme conditions such as in liquid nitrogen (−196 °C) or at a temperature of 900 °C. Thus, from a structural viewpoint, we believe that our graphene sponge may be likened to a 3D cross-linked polymer, but with the graphene sheets behaving as the cross-linked building block (monomer) as in the case of thermoset polymers where the curing process transforms the linear polymers into a 3D monolithic structure through the cross-linking process [16] , [17] , [26] . We will provide evidence that the uncompressed graphene sponge is homogenous and nearly isotropic, which is important since the direction of gravity during synthesis could conceptually provide important and large differences in properties for the axial direction (the gravity d irection during synthesis in a cylinder) and the radial direction of this cylinder. An important question is whether or not a largely isotropic, additive-free graphene sponge can be highly elastically deformable. In fact, Qiu et al . [7] have shown that freeze casting the partly reduced graphene oxide could result in highly anisotropic cork-like structures that provide large stroke elastic deformability (when sponge assembly uses columnar growth of ice), and that much less ordered porous graphene monoliths that made by chemical vapour deposition and self-gelation were not highly elastic. In principle, freeze-cast graphene aerogels might also be overall isotropic if anisotropic domains are randomly connected with an optimized control of the ice template [7] . Figure 1d shows typical cross-sectional scanning electron microscopy (SEM) images of our sponge containing about 99.9% or higher void volume (depending upon the density of the sponge walls). To see deep inside a sponge’s interior, a 3D image was obtained by stacking optical images acquired during sequential laser-ablation of the 15-μm slices of the sponge ( Supplementary Movie 1 and Supplementary Fig. 5 ). These imaging results indicate that the sponge consists of a 3D array of interconnected micron-scale voids, which are partially tiled in a disordered manner by graphene sheets (see also Supplementary Figs 6 and 7 , which provide SEM micrographs of a planar sponge surface containing orthogonal radial and axial directions). The full mechanism to form such large size pores needs more understanding. The ‘axial’ direction refers to the gravity direction (the axial direction of the initially cylinder shaped aerogel) and the radial directions are orthogonal to the axial direction. Raman spectra obtained for different polarization directions about two different incident laser beam directions (axial and radial) are consistent with a nearly isotropic structure for the non-compressed structure ( Fig. 2a and Supplementary Fig. 8 ). During compression up to 90% strain, the sponge becomes increasingly anisotropic, because of slight strain-induced alignment of the graphene sheets perpendicular to the strain direction. For 0% strain the ratio of maximum-to-minimum G-band intensity is closer to unity for light propagating in the axial direction (0.976) than in the radial direction (0.894) and both ratios slightly decrease upon compression to 90% strain (to 0.905 and 0.857, respectively). Importantly, the structure of our graphene sponge completely recovered when the compressive stress was released, indicating remarkable structural stability even for such extreme strains. This high structural stability is also supported by its fully recoverable and near-direction-invariance of various properties under cycling tests: electrical conductivity in the compression direction for 0–90% strain ( Supplementary Fig. 9 ), thermal expansion coefficient ( Supplementary Fig. 10 ), Young’s modulus ( Supplementary Fig. 11 ), SEM and Fast Fourier Transformation images ( Supplementary Fig. 6 ), and the below described Poisson’s ratio ( Supplementary Fig. 12 ). 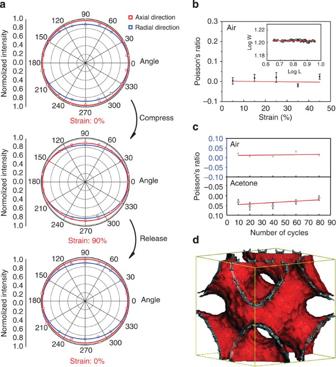Figure 2: Sponge anisotropy and Poisson’s ratios. (a) The normalized intensity of the Raman G band (for 633 nm excitation) as a function of polarization angle for a strain cycle between 0 strain and 90% strain and back to 0% strain. Open red squares (and red fitting curves) are for light propagating in the axial direction and strain applied in the radial direction and the open blue squares (and the blue fitting curves) are for light propagating in the radial direction and strain applied in the axial direction. (b) The Poisson’s ratio in air as a function of applied strain in the axial direction. The data points are the Poisson’s ratios obtained in 10% strain intervals by least squares fit of the logWversus logLdata for these intervals that is shown in the inset (which is a plot of logWversus logL, whereWandLare sample dimensions in the width and compression directions). The red lines in both the figure and the inset are linear least square fits of all of the respective data points. The error bars of Poisson’s ratio at each strain are obtained as the s.e. from the least squares fit of the logWversus logLdata shown in the inset for each such strain. (c) Poisson’s ratio as a function of number of compression and release cycles along the axial direction. The blue diamonds (top) and black stars (bottom) are Poisson’s ratios when the sponge is in air and in acetone, respectively. The error bars indicate the s.e. obtained from the fitted curve when we calculate the Poisson’s ratio by using the logWversus logLmethod. (d) The Schwartzite model for sp2-carbon phases used for the Poisson’s ratio modelling, where the illustrated phase has a cell parameter ofa=2.38 nm. Figure 2: Sponge anisotropy and Poisson’s ratios. ( a ) The normalized intensity of the Raman G band (for 633 nm excitation) as a function of polarization angle for a strain cycle between 0 strain and 90% strain and back to 0% strain. Open red squares (and red fitting curves) are for light propagating in the axial direction and strain applied in the radial direction and the open blue squares (and the blue fitting curves) are for light propagating in the radial direction and strain applied in the axial direction. ( b ) The Poisson’s ratio in air as a function of applied strain in the axial direction. The data points are the Poisson’s ratios obtained in 10% strain intervals by least squares fit of the log W versus log L data for these intervals that is shown in the inset (which is a plot of log W versus log L , where W and L are sample dimensions in the width and compression directions). The red lines in both the figure and the inset are linear least square fits of all of the respective data points. The error bars of Poisson’s ratio at each strain are obtained as the s.e. from the least squares fit of the log W versus log L data shown in the inset for each such strain. ( c ) Poisson’s ratio as a function of number of compression and release cycles along the axial direction. The blue diamonds (top) and black stars (bottom) are Poisson’s ratios when the sponge is in air and in acetone, respectively. The error bars indicate the s.e. obtained from the fitted curve when we calculate the Poisson’s ratio by using the log W versus log L method. ( d ) The Schwartzite model for sp 2 -carbon phases used for the Poisson’s ratio modelling, where the illustrated phase has a cell parameter of a =2.38 nm. Full size image Near-zero Poisson’s ratio in both directions Poisson’s ratio ( ν ij ) is defined as ν ij =− ε j / ε i , where ε j is the j-direction lateral strain resulting from an applied longitudinal strain ε i (refs 27 , 28 , 29 , 30 , 31 ). Ordinary rubbers exhibit Poisson’s ratios of ~0.5. Cork does have a near-zero Poisson’s ratio when compressed in the axial direction, which makes it easy to insert and remove a cork from a wine bottle [32] . However, cork is not an elastomer, so large applied strains cause irreversible plastic deformation. Though a small Poisson’s ratio was noted for very low-density elastomeric carbon aerogels made by templating a ZnO rod array with carbon to make an array of short, micron-diameter hollow rods, neither Poisson’s ratio measurements nor characterization of anisotropy were reported [33] . A negative Poisson’s ratio has been reported for an aerogel based on graphene cell walls coated with CNTs [2] . Also, measurements for a single wall nanotube aerogel show that near-zero Poisson’s ratios for 0–60% strain in one direction [34] . In contrast to the largely near-zero strain-invariant Poisson’s ratios that we will describe, extreme sensitivity of Poisson’s ratio to applied tensile strain has been reported for CNT sheets, where the Poisson’s ratio continuously changes from about −0.5 to 0.3 during in-plane tensile strains of only 1.4% or smaller [35] . Perhaps the largest reported strain dependence of Poisson’s ratio has been described for highly anisotropic, fibrillated polytetrafluoroethylene, where ν was found to decrease from 0 to −14 in a true strain range of 0.03 (ref. 36 ). We investigated the dependence of the graphene sponge’s Poisson’s ratio on applied compressive strain in both the axial and radial directions by recording movies during deformation to measure sponge width ( W ) as a function of the sponge length ( L ) along the compression direction. Using the definition for infinitesimal strains, the Poisson’s ratio is found (for small strain changes around a giant applied strain) as the negative slope of log W versus log L (inset of Fig. 2b ). Importantly, the Poisson’s ratios were close to zero (in air and when immersed in acetone) both for compression in the axial ( Fig. 2b,c ) and radial directions ( Supplementary Figs 12 and 13 ). Furthermore, during each compression and release cycle, the Poisson’s ratio remained near zero and showed little strain dependence ( Fig. 2b ). This near-zero Poisson’s ratio was reproducible for all the over 80 measured compression and release cycles in air/acetone for both compression directions ( Fig. 2c and Supplementary Fig. 13 ). In contrast with these results, carbon foams investigated by Li et al . [37] , which are produced from blown anisotropic pitch, have a predicted Poisson’s ratio that strongly depends upon foam density, and reaches large observed values (~0.3) for low foam densities. Such blown, pitch-derived carbon foams might be most simply viewed as an array of hollow spheres—if you compress the spheres they laterally expand, thereby providing large Poisson’s ratios. Similarly, if compression of our graphene sponges had resulted in highly preferential alignment of the graphene planes perpendicular to the compression direction, a large positive Poisson’s ratio would be expected. However, Raman measurements during compression show (even for 90% compressive strain) that very little anisotropy is introduced into the alignment of the graphene planes ( Fig. 2a and Supplementary Fig. 8 ). This Raman data indicate that massive sidewall buckling is occurring during 90% compressive strain and suggests that this bucking is critically important for explaining the existence of near-zero Poisson’s ratios to extreme strains (like the case for enormously smaller deformations for cork in only one direction). The low sponge density at even 98% compression (~50 mg cm −3 ), means that buckled sponge sidewalls largely do not contact to provide lateral expansion. Since the elastic properties of an isotropic material depend on only three independent constants, which can be chosen as the Poisson’s ratio ( ν ), the bulk modulus ( B ) and the shear modulus ( G ) (or the Young’s modulus, Y , where Y =2 G (1+ ν ) for isotropic materials), we can derive G / B and Y / B for ν =0 from the isotropic material equation (1) [38] : This provides G / B =3/2 and Y / B =3 over the large-strain range that we have above investigated. Although Poisson’s ratio is ordinarily defined for mechanical deformations in which the sample composition is invariant, we have here extended results to sponge deformation when immersed in a liquid with a newly defined ‘skeletal Poisson’s ratio’. This skeletal Poisson’s ratio describes changes in the graphene sponge dimensions as the imbibed liquid is extruded out and then reabsorbed when the compression is removed. Using the same type of analysis as for the graphene sponge in air, we obtained essentially identical results to those obtained in air for a graphene sponge containing 71,000 wt% of imbibed acetone. For measurements recorded between 0 and ~50% compressive strain in the axial direction, the skeletal Poisson’s ratio is nearly zero (lower half of Fig. 2c ) and did not change over the measured 80 cycles of imbibing and releasing nearly 100% of the compressed volume. Similarly, near-zero skeletal Poisson’s ratios were obtained for compression along the radial direction, and remained unchanged during cycling (lower half of Supplementary Fig. 13 ). The largely isotropic, near-zero Poisson’s ratio over giant strain ranges has important consequences. First, if a material laterally expands or contracts (due to positive or negative Poisson’s ratios, respectively), friction at the compressing platens will cause non-uniform lateral deformation—the compressed sponge would balloon outwards for a positive Poisson’s ratio or collapse inwards for a negative Poisson’s ratio (relative to the constrained lateral dimensions at the platens) [29] . Neither of these effects, which could limit the strain range for reversible compression, are noticeable for either our neat or liquid-imbibed sponges where Poisson’s ratio is characterized. Second, if the sponge had a normal positive Poisson’s ratio of about 0.3 that was isotropic about the compression axis, the fraction of liquid volume extruded from the sponge by an uniaxial strain Δ L / L would be reduced from Δ L / L to Δ L / L (1–2 ν ) or by 60%. Since the disordered graphene sponge has a somewhat similar sp 2 -carbon tiled open-pore structure to that of the cubic Schwartzite phase [39] shown in Fig. 2d , we investigated (see Supplementary Methods for details) whether the Schwartzite structure would possess a near-zero Poisson’s ratio. This Schwartzite phase has average Poisson’s ratios of −0.040, 0.080 and 0.128 for compression along the (100), (110) and (111) directions, and an average Poisson’s ratio (considering all compression and lateral directions) of between 0.040 (Voigt average) and 0.056 (Reuss averages; refs 40 , 41 ). Such averaging of non-zero Poisson’s ratios for microscopic elements to provide a near-zero macroscopic average likely also occurs for our materials. Super compressive elasticity The remarkable compressive elasticity of the graphene sponge during large-strain cycling in air and liquid are further demonstrated in the results of Fig. 3a,b and Supplementary Figs 7,14,15 . Substantially reversible deformation was retained even for a compression ratio (ratio of initial to final length) of 50 (corresponding to ~98% strain) shown in the inset of Fig. 3a and Supplementary Movie 2 , which appears to be largest isotropic elastic deformability reported so far for any form of carbon [2] , [4] , [7] , [9] , [42] . 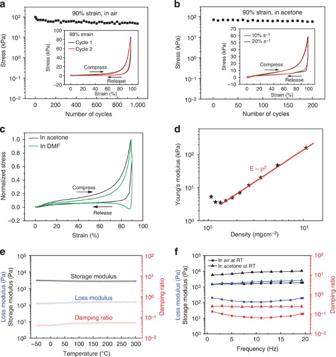Figure 3: The mechanical behaviour when compressed along the axial direction. (a) The compressive stress to reach 90% strain at an engineering strain rate of 40% strain s−1is plotted as a function of cycle number for 1,000 cycles in air. The inset shows the reversibility of stress–strain curves for two successive cycles in air (black and red curves, respectively) up to a compressive strain of 98%. (b) The compressive stress needed to reach 90% strain at an engineering strain rate of 20% strain s−1is plotted as a function of cycle number for 200 cycles. The inset shows stress–strain cycles in acetone up to 90% strain for engineering strain rates of 10% strain s−1(red line) and 20% strain s−1(black line). (c) Comparison of stress–strain cycles up to 90% strain in acetone (black curve) and in DMF (green curve) at an engineering strain rate of 20% strain s−1. The stresses are normalized to the maximum stress applied. (d) The dependence of Young’s modulus on the density (ρ) realized during a compression/release cycle. The red line corresponds toY=Aρn, where A is a constant andn=1.898±0.041. (e) The temperature dependence of storage modulus (black), loss modulus (blue) and damping ratio (red) from DMA measurements at 10 Hz between −50 and 300 °C. (f) The frequency dependence of storage modulus (black), loss modulus (blue) and damping ratio (red) that was obtained from DMA measurements for the graphene sponge at RT (room temperature) in both air and acetone. Figure 3: The mechanical behaviour when compressed along the axial direction. ( a ) The compressive stress to reach 90% strain at an engineering strain rate of 40% strain s −1 is plotted as a function of cycle number for 1,000 cycles in air. The inset shows the reversibility of stress–strain curves for two successive cycles in air (black and red curves, respectively) up to a compressive strain of 98%. ( b ) The compressive stress needed to reach 90% strain at an engineering strain rate of 20% strain s −1 is plotted as a function of cycle number for 200 cycles. The inset shows stress–strain cycles in acetone up to 90% strain for engineering strain rates of 10% strain s −1 (red line) and 20% strain s −1 (black line). ( c ) Comparison of stress–strain cycles up to 90% strain in acetone (black curve) and in DMF (green curve) at an engineering strain rate of 20% strain s −1 . The stresses are normalized to the maximum stress applied. ( d ) The dependence of Young’s modulus on the density ( ρ ) realized during a compression/release cycle. The red line corresponds to Y = Aρ n , where A is a constant and n =1.898±0.041. ( e ) The temperature dependence of storage modulus (black), loss modulus (blue) and damping ratio (red) from DMA measurements at 10 Hz between −50 and 300 °C. ( f ) The frequency dependence of storage modulus (black), loss modulus (blue) and damping ratio (red) that was obtained from DMA measurements for the graphene sponge at RT (room temperature) in both air and acetone. Full size image During 1,000 compression cycles in air to 90% strain ( Fig. 3a ) our graphene sponge shows relatively minor decrease in the stress required to deform it to this strain level. These results are for an engineering strain rate of 10% strain s −1 (normalized to the uncompressed sponge length, which increases with increasing strain up to 100% strain s −1 when normalized to the instantaneous sponge length). During compression up to 98% strain ( Fig. 3a ) the sponge can reversibly absorb 8.3 J g −1 of mechanical energy, of which 5.4 J g −1 is dissipated as heat during the stress–strain cycle. Note in Fig. 3a that most of this mechanical energy conversion occurs in the engineering strain range between 60 and 98%. The structural stability of our graphene sponge is further supported by electrical resistance measurements during compression/release cycles ( Supplementary Fig. 16a ), which shows that there is little change in the uncompressed electrical resistance after 100 cycles to 80% strain and the dependence of electrical resistance and gravimetric conductivity on strain is the same during compression and compression release. Remarkably, our graphene sponge can reversibly undergo large-strain deformation (up to 90%) in which liquids (such as acetone, ethanol, N , N -dimethylformamide (DMF), silicon oil, and paraffin oil) are reversibly absorbed and then discharged by subsequent compression ( Fig. 3b,c ; Supplementary Fig. 15 ; and Supplementary Movie 3 ). Interestingly, there is no noticeable change in the compressive stress needed to extrude a low-viscosity liquid (like acetone) from the sponge, even when strain rate was doubled to an engineering strain rate of 20% strain s −1 , and a true strain rate of up to 200% strain s −1 ( Fig. 3b inset). However, the identical comparison for a higher viscosity imbibed liquid (DMF) shows that the stress required to achieve 90% compressive strain increases when the strain rate is doubled ( Supplementary Fig. 15 ). When acetone is reabsorbed during sponge elongation ( Fig. 3b inset), the measured stress exhibits some dependence on strain rate for strains between 90 and 80%. More surprising, the measured stress for a sponge containing DMF dips below zero for high axial-direction strains ( Fig. 3c and Supplementary Fig. 15 insets). These below-zero measured stresses result from the inability of liquid absorption to keep up with the giant true strain rate, owing to DMF’s high viscosity (0.796 versus 0.316 cP for acetone at 25 °C). The sponge therefore adheres to the platens of the stress–strain measuring apparatus, causing the expected compressive stress to temporarily switch to a tensile stress. Some differences in stress do exist between experimental results for axial compression ( Fig. 3b inset, Supplementary Fig. 15a inset, Supplementary Fig. 17 ) and radial compression ( Supplementary Fig. 15b inset, Supplementary Fig. 18 ), which likely result from differences in sample dimensions, density and porosity. In contrast with this remarkable giant stroke elastic deformability of our sponges in compression (up to 98% compressive strain), they fail by a brittle fracture in air at below 5% strain when uniaxially stretched ( Supplementary Fig. 19 ). The reason is likely twofold. First, since the Poisson’s ratio is near zero, tensile strain decreases the sponge density (rather than increases it) so there are fewer (but longer mechanical) struts supporting the load. Second, as for many materials, tension causes defects (like cracks) to propagate. The dependence of Young’s modulus on the density realized during extreme sponge compression ( Supplementary Fig. 20 ) is shown in Fig. 3d . Except for the initial small strains, where there is uncertainty in the applied strain, the Young’s modulus depends approximately quadratically on sponge density ( ρ ) over a 10-fold density range. Remarkably, this power dependence of Young’s modulus on ρ , while the sponge is being compressed to ~10% of initial height (that is, Y = Aρ n , where A is a constant and n =1.892±0.041), is within experimental error of the n =2.21±0.23 power dependence of modulus obtained for small-strain deformation of sponges having different initial densities ( Supplementary Fig. 11 ). A quadratic dependence of low strain modulus on initial aerogel density has been reported for diverse materials [7] , [30] , [34] , [43] , [44] , and is generally associated with a low-density, open-cell architecture [43] , [44] , [45] . These sponge results are consistent with efficient load transfer to aerogel struts (presently graphene sheet cell walls) that undergo transverse-beam-bending [43] , [44] . That about the same quadratic power dependence on density results for giant compressions is apparently new for any aerogel, and suggests efficient load transfer to sponge sidewalls that are undergoing reversible buckling. We observe that remarkable reversible compressive elasticity to giant strains even at extremely low and high temperatures (from −196 to 900 °C). Supplementary Fig. 21a and Supplementary Movie 4 show compression and release in liquid N 2 , where the sponge reversibly absorbs and extrudes liquid nitrogen. Similar large-strain elasticity was observed at 900 °C in argon atmosphere ( Supplementary Fig. 21b and Supplementary Movie 5 ). While annealing the graphene sponge at 900 °C in argon, which is much longer than the time at this temperature required for the compressibility test (~10 min), increased the carbon content from 86.30 to 92.41 wt%, decreased the oxygen content from 11.86 to 6.59 wt% and decreased the hydrogen content from 1.84 to 1.00 wt%, the SEM images in Supplementary Fig. 22 show that hour-long thermal annealing at 900 °C does not noticeably change sponge structure. The above high-strain uniaxial elasticity over such a wide temperature range has apparently not been reported for any other compressively elastomeric material, for instance, commercial silicone rubber becomes brittle at −55 °C and degrades above 300 °C (ref. 46 ). Dynamic mechanical analysis Notably, the material also demonstrates rather stable viscoelastic temperature- and frequency- invariant stability, reversible deformation and fatigue resistance. DMA measurements of the sponge’s viscoelastic properties in air and liquids show that the origin of sponge compressive elasticity is enthalpic, rather than the entropic elasticity found for ordinary rubbers [10] , [11] . As a consequence, in contrast to the conventional elastomers like silicone rubber, the sponge’s storage and loss moduli depend relatively little on temperature (−50 to 300 °C in air for Fig. 3e ) or frequency (1–20 Hz at room temperature in air and acetone for Fig. 3f , and at 300 °C in air for Supplementary Fig. 23 ) [46] . DMA measurements in air at 300 °C show negligible change in storage and loss moduli during 100,000 cycles ( Supplementary Fig. 24 ). Since these cycles subject the sponge to 300 °C in air for 1.4 h, these negligible changes in storage and loss moduli indicate the remarkable thermal stability of the sponge, which is also evident from thermal gravimetric measurements and combustion flame tests ( Supplementary Fig. 25 and Supplementary Movie 6 ). At room temperature, similar stability of storage and loss moduli were observed during 100,000 compression cycles in both air and acetone ( Supplementary Fig. 26 ), indicating an excellent reversible deformation and fatigue resistance even in fluid for this superelastic graphene material. With the unique structure and combination of a wide range and temperature- invariant properties, together with its low density and close to 100% porosity (see below), this material should find some interesting and novel applications when multifold properties are required. Indeed, the ability of the graphene sponge to reversibly absorb and discharge liquids during compression ( Supplementary Movie 7 ) and its strong hydrophobicity (water contact angle 135°) suggests its possible application for environmental cleanup and convenient liquid transfer. This possibility is made particularly attractive by its high cycle life ( Fig. 3b ), the short times to achieve 90% liquid extrusion and complete reabsorption for even viscous liquids (4.5 s for DMF in Fig. 3c ), and the high realized weight ratio of absorbed liquid ( Fig. 4a,b and Supplementary Fig. 27 ). For example, our graphene sponge can reversibly absorb and extrude up to 1,010 times its weight of pump oil, which is 3.2 times higher than for the highest performing solid absorbent previously reported for pump/engine oil ( Fig. 4a ) [2] , [9] . Fig. 4b shows that the percent increase in sponge weight is approximately linearly dependent on the liquid density, which is consistent with past studies [2] , [9] . Note, the utilization of the porosity of our graphene material is very efficient in all cases, going up to >99% and close to the 100% theoretical limit. The volume ratio of absorbed liquid to the approximate graphene volume within the sponge (approximating the graphene density as 1.7 g cm −3 ) was also large, reaching uptake ratios of 198,000% for pump oil ( Supplementary Fig. 27 ). The possible liquid transfer ability of this material is demonstrated in Supplementary Movie 7 , where when the saturated graphene material is pressed, the absorbed liquid can be compressed out almost completely and the material can be reused without any damage. This absorption/release process is highly repeatable, and no change or degrading was observed even after hundreds of times of cycles, indicating the sponge’s high structural stability. No visible extrusion or leaking of liquid were observed during this process. The high absorption ability and excellent absorption/release cycling property indicate that it can be used for absorption and transfer of various liquid materials, environmental cleanup and medical device applications and so on. 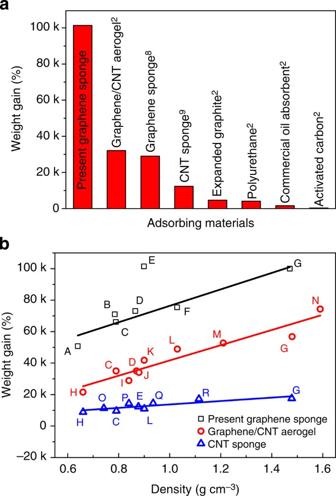Figure 4: The liquid absorption capabilities of the graphene sponge. (a) The liquid adsorption capacity in (percent weight gain during liquid absorption) of the graphene sponge for pump oil, compared with that of other absorbents2,9for either pump or engine oil. (b) Linear least squares fit lines for the relationship between the liquid adsorption capacity and the density of the absorbed liquid for the present sponges (black line), graphene aerogels containing CNT coated cells2(red line) and CNT sponges9(blue line). Comparison of the correlation lines for these three materials show the major performance advantage of the present graphene sponge. The data points are for absorption of: A, petroleum ether; B, acetone; C, ethanol; D, toluene; E, pump oil; F,N-methyl pyrrolidone; G, chloroform; H,n-hexane; I, crude oil; J, motor oil; K, vegetable oil; L, 1,4-dioxane; M, 1-butyl-3-methylimidazolium tetrafluoroborate; N, carbon tetrachloride; O, gasoline; P, diesel oil; Q, DMF; and R, ethylene glycol. Figure 4: The liquid absorption capabilities of the graphene sponge. ( a ) The liquid adsorption capacity in (percent weight gain during liquid absorption) of the graphene sponge for pump oil, compared with that of other absorbents [2] , [9] for either pump or engine oil. ( b ) Linear least squares fit lines for the relationship between the liquid adsorption capacity and the density of the absorbed liquid for the present sponges (black line), graphene aerogels containing CNT coated cells [2] (red line) and CNT sponges [9] (blue line). Comparison of the correlation lines for these three materials show the major performance advantage of the present graphene sponge. The data points are for absorption of: A, petroleum ether; B, acetone; C, ethanol; D, toluene; E, pump oil; F, N -methyl pyrrolidone; G, chloroform; H, n -hexane; I, crude oil; J, motor oil; K, vegetable oil; L, 1,4-dioxane; M, 1-butyl-3-methylimidazolium tetrafluoroborate; N, carbon tetrachloride; O, gasoline; P, diesel oil; Q, DMF; and R, ethylene glycol. Full size image The highly elastic structure of the graphene sponge can be maintained even when functional materials are inserted before or after synthesis with this sponge as a supporting framework or template. For example, a magnetically driven magnetostrictive actuator was made by infiltrating Fe 3 O 4 particles into the as-synthesized graphene sponge ( Supplementary Fig. 28 ). When driven by a 15-mT (150 Gauss) magnetic field, a sponge containing 30 wt% loading of Fe 3 O 4 nanoparticles provided 60% stroke ( Supplementary Figs 28,29 ). This simple device exhibits reversible magnetic actuation ( Supplementary Movie 8 ) without any degradation during 1,000,000 stroke cycles to ~10% actuator strain, as well as actuation at up to 100 Hz. Similarly, other functional materials may be inserted in the same way to obtain multifunctional materials with super elasticity. In summary, we fabricated and characterized a novel, additive-free bulk graphene sponge that provides a host of surprising properties. First, these sponges exhibit reversible superelastic properties at temperatures between −196 (for liquid nitrogen) and 900 °C (in inert atmosphere), and recover up to 98% compression in air and 90% in liquids, demonstrated by thousands of compression/releasing cycles with giant strains. Second, independent of the compression direction, these nearly homogenous sponges consisting of 3D and randomly chemically bonded graphene sheets provide a Poisson’s ratio and a skeletal Poisson’s ratio that is near-zero and substantially independent of strain, even when giant compressive strains are applied in air or for liquid-imbibed sponges. Third, these graphene sponges can absorb up to 1,010 times their weight of a liquid and then reversibly and repeatedly discharge the liquid in seconds when compressed. With these unique combined properties combing both the characteristic properties from both rubber and cork in wide temperature range, together with its over 99.9% porosity, it is highly possible to develop various high-end applications where multifold functions are demanded simultaneously. Note, all these excellent properties are above both the high chemical and thermal stability of graphene (carbon) materials, which should make this material highly desirable for many harsh environment applications where such multifold functions are required. Also, this indicates that assembling the wonderful 2D graphene sheets into bulk 3D state may generate novel materials with unprecedented properties. It is also possible to engineer and obtain some other novel and exotic materials using other 2D building blocks widely available recently using similar approach, if they are assembled into the 3D mode where the individual 2D unit intrinsic properties are kept. To this end, these materials are expected to have broad implications for novel material design and their applications. Fabrication of the graphene sponge The starting material, GO, was prepared by the oxidation of natural graphite powder using a modified Hummers method. The graphene sponge was fabricated by an in situ solvothermal process that uses ethanol as the solvent for low concentrations of GO sheets (having ~20 to 50 μm lateral dimension). Initial GO ethanol solutions were made from aqueous GO solutions (~1.50 mg ml −1 ) by replacing water with ethanol using isopycnic differential centrifugation at 12,000 r.p.m. This exchange was repeated six times (each time using ~30 ml ethanol to dilute ~1 mg GO) to ensure essentially complete exchange with ethanol. The low concentration GO ethanol solution (0.20–5.00 mg ml −1 ) was then solvothermally treated in a Teflon-lined autoclave at 180 °C for 12 h to form an intermediate solid, which has about 1/3 to 1/2 of the GO solution volume before the solvothermal reaction. The use of ethanol as a solvent was important, since graphene aerogels made directly from water solution did not have the desired extreme rubber-like elasticity. The size of the GO flakes in the starting material has a major impact on the properties of the final graphene sponge—use of the above large size graphene flakes enhanced mechanical robustness and reversible large-strain elasticity. After the solvothermal reaction, the ethanol-filled sponge was carefully removed from the autoclave and fully immersed in a mixture of acetone and ethanol (1:1 by volume). Then water was slowly added to the system until the sponge was fully immersed in water, thereby enabling the exchange of the ethanol absorbed inside of the sponge with water. Then ~1/3 of the solvent volume was slowly removed by decanting. Thereafter, water was added to again cover the sponge. This step was then repeated about 15–20 times. It usually takes ~6 h for each cycle and up to 5–7 days for the whole process. After the solvent exchange process, the water-filled sponge was freeze-dried to remove the remaining water absorbed in the sponge. Finally, the cylindrically shaped sponge was annealed at 400 °C for an hour in argon to obtain the final compressively elastomeric graphene sponge. For specific measurements, these graphene sponges can be easily cut using a laser (450 nm, 2 W) into desired shapes and sizes. Various sample sizes, with volumes up to hundreds of cubic centimetres, were produced by varying the dimensions of the solvothermal reactor. Two directions of the sample are defined for the convenience of measurement. The ‘axial’ direction refers to the gravity direction (the axial direction of the cylinder shaped sample) when the graphene sponge is made in the autoclave. The direction perpendicular to the axial direction is named as the ‘radial’ direction. How to cite this article: Wu, Y. et al . Three-dimensionally bonded spongy graphene material with super compressive elasticity and near-zero Poisson’s ratio. Nat. Commun. 6:6141 doi: 10.1038/ncomms7141 (2015).